RETRACTED ARTICLE: Precise determination of graphene functionalization byin situRaman spectroscopy The verification of a successful covalent functionalization of graphene and related carbon allotropes can easily be carried out by Raman spectroscopy. Nevertheless, the unequivocal assignment and resolution of individual lattice modes associated with the covalent binding of addends was elusive up to now. Here we present an in situ Raman study of a controlled functionalization of potassium intercalated graphite, revealing several new bands appearing in the D-region of the spectrum. The evolution of these bands with increasing degree of functionalization from low to moderate levels provides a basis for the deconvolution of the different components towards quantifying the extent of functionalization. By complementary DFT calculations we were able to identify the vibrational changes in the close proximity of the addend bearing lattice carbon atoms and to assign them to specific Raman modes. The experimental in situ observation of the developing functionalization along with the reoxidation of the intercalated graphite represents an important step towards an improved understanding of the chemistry of graphene. The wet-chemical exfoliation of graphite intercalation compounds (GICs) and the subsequent treatment with electrophiles is one of the most potent methods for covalent graphene functionalization [1] , [2] , [3] , [4] , [5] . For this purpose, graphite is typically activated by saturation doping with potassium to reach the highest stage I intercalation level with a crystalline K to C ratio of 1:8 (refs 6 , 7 ). In the subsequent covalent binding step, a single electron transfer to the electrophile (for example, alkyl halide [8] or diazonium compound [4] ) takes place and, after halide− or N 2 elimination, the intermediately formed organic radical attacks the conjugated π -system of the graphenide upon the formation of sp 3 centres in the carbon lattice [9] , [10] , [11] , [12] . The degree of functionalization (DOF) depends on the reduction potential of the electrophile and if this is low enough, almost all negative charges of the graphenide can be quenched [13] , [14] . In our recent work, we were able to provide a simple and efficient procedure for the quantitative discharging of reduced graphites using benzonitrile as trapping reagent that allows for the synthesis of defect-free graphene from graphenide solutions [6] . The verification of the successful covalent functionalization and the determination of the quality of exfoliated graphene can be obtained by Raman spectroscopy that serves as the most important characterization tool for the analysis of graphene-based materials [15] , [16] , [17] , [18] . It is a nondestructive technique, allowing for unravelling the interaction between individual graphene sheets and functional groups. Raman spectroscopy and, in particular, statistical Raman microscopy [9] can also be used to analyse the doping effects [19] , [20] , strain [21] , oxidation and sample quality [22] , [23] , [24] , molecular functionalization [25] and number of layers [26] . For this purpose, characteristic changes of the most prominent Raman modes, namely, the D, G and 2D modes are the most significant indicators [15] . However, a graphitic framework containing lattice embedded sp 3 carbon atoms—generally termed as sp 3 defects—gives rise to additional Raman modes [15] . Moreover, recent work predicted the presence of additional Raman bands for hydroxylated graphene [22] that have already been observed in graphene oxide (GO) samples [27] . In addition, first approaches for the quantification of sp 3 defects have been reported [28] , [29] . Based on these considerations we have developed a geometrical model revealing the DOF θ as ratio of the basal sp 3 / sp 2 carbon atoms by the use of scanning Raman spectroscopy for statistical analysis [9] , [30] . However, the information obtained from Raman spectroscopy is only valid for interdefect distances of ∼ 3 nm (refs 28 , 29 ) and the corresponding θ <0.5% (refs 9 , 30 ). Therefore, functionalized graphene derivatives like polyhydrogenated graphene [31] , [32] or graphene oxide [33] , [34] still cannot be addressed. In those cases, the D, G and 2D modes appear as very broad and poorly resolved features [18] hiding the individual contributions from the individual lattice vibrations [35] , [36] . The unequivocal assignment and resolution of individual lattice modes introduced by covalent binding was elusive and remained a major challenge in graphene chemistry. Tackling this problem would require the in situ spectroscopic monitoring of the reaction progress before the defect-induced broadening of the Raman modes in highly functionalized samples prevents any line shape analysis and a detailed understanding of the correlation between defect-related Raman modes and the atomic structure of the addend carrying neighbourhood in the covalent adduct. Here we report a comprehensive study involving in situ Raman spectroscopy supported by quantum mechanical calculations where we have successfully solved the challenges pointed out above. As model reaction we have chosen the hydrogenation of reduced graphite [32] with H 2 O and compared it with the corresponding exposure to H 2 and O 2 . Next to the very precise characterization of the covalently functionalized graphene by an unambiguous assignment of the lattice vibrations, we are furthermore able to provide profound mechanistic information on the underlying covalent addition chemistry. Our results are of fundamental importance for any laboratory investigating the chemistry and materials design of graphene, graphene composites and other functional synthetic carbon allotropes. In situ monitoring of the chemical functionalization The setup of the in situ Raman monitoring of the reaction of defect free KC 8 crystals with H 2 O, H 2 and O 2 is presented in Fig. 1a . This high-end system enables an unprecedented precise reaction control since a focused scenario consisting of the two reaction partners is provided. In this setup, the partial pressure of the volatile component at the solid/gas interphase is the only parameter that is varied. The in situ Raman setup is equipped with a laser probe (excitation wavelength 514 nm) that allows for the spectroscopic monitoring of the reaction and the detection of the stepwise evolution of functionalization-related Raman modes. The required stage I GIC was prepared under argon atmosphere [6] . The successful and clean formation of KC 8 was confirmed by Raman spectroscopy and by X-ray diffraction (XRD) analysis ( Supplementary Fig. 1 ). After controlled exposure to H 2 O vapour we were able to monitor the early stages of the reaction (low degree of addition) associated with a mild surface hydrogenation ( Fig. 1b ). In Fig. 1c , the evolution of the Raman spectra of a fully doped GIC ( n K + C 8 n − ) is presented upon extended exposure to H 2 O vapour. The gradual growth of distinct modes becomes apparent. 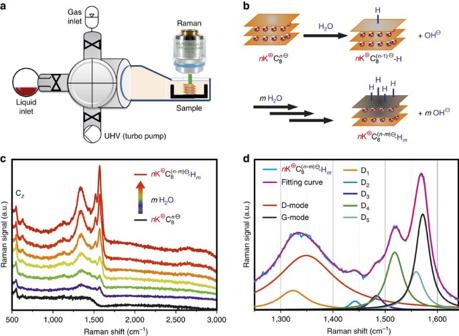Figure 1: Raman setup andin situspectroscopic monitoring of the covalent functionalization of KC8. (a) Schematic illustration of the setup for the controlled reaction of KC8with liquid and/or gaseous reagents under ultra-high vacuum conditions. The reaction progress is monitored byin situRaman spectroscopy. (b) Scheme of the model reaction: defect-free stage I GIC (nK+C8n−) was exposed to H2O vapour. After the initiation of the reaction, hydrogenated graphene is formed. (c) Evolution of the Raman spectra fromnK+C8n−(black, bottom) to hydrogenatednK+C8(n-m)−-Hm(red, top) in the first stages ofsp3defect site formation in the crystal. (d) Raman fingerprint ofnK+C8(n-m)−-Hmafter addend binding andsp3defect site formation within the graphene lattice. The D- and G-line region (1,200–1,700 cm−1) contains 7 components: graphiticE2gG mode (∼1,575 cm−1) and defect activated D mode (∼1,340 cm−1), and five additional defect modes discovered for the first time in this study, namely, D1(∼1,325 cm−1), D2(∼1,442 cm−1), D3(∼1,483 cm−1), D4(∼1,518 cm−1) and D5(∼1,559 cm−1), that originate from carbon bond vibrational coupling deviations in the vicinity of thesp3defect site. Figure 1: Raman setup and in situ spectroscopic monitoring of the covalent functionalization of KC 8 . ( a ) Schematic illustration of the setup for the controlled reaction of KC 8 with liquid and/or gaseous reagents under ultra-high vacuum conditions. The reaction progress is monitored by in situ Raman spectroscopy. ( b ) Scheme of the model reaction: defect-free stage I GIC ( n K + C 8 n − ) was exposed to H 2 O vapour. After the initiation of the reaction, hydrogenated graphene is formed. ( c ) Evolution of the Raman spectra from n K + C 8 n − (black, bottom) to hydrogenated n K + C 8 ( n - m )− -H m (red, top) in the first stages of sp 3 defect site formation in the crystal. ( d ) Raman fingerprint of n K + C 8 ( n - m )− -H m after addend binding and sp 3 defect site formation within the graphene lattice. The D- and G-line region (1,200–1,700 cm −1 ) contains 7 components: graphitic E 2g G mode ( ∼ 1,575 cm −1 ) and defect activated D mode ( ∼ 1,340 cm −1 ), and five additional defect modes discovered for the first time in this study, namely, D 1 ( ∼ 1,325 cm −1 ), D 2 ( ∼ 1,442 cm −1 ), D 3 ( ∼ 1,483 cm −1 ), D 4 ( ∼ 1,518 cm −1 ) and D 5 ( ∼ 1,559 cm −1 ), that originate from carbon bond vibrational coupling deviations in the vicinity of the sp 3 defect site. Full size image After a few minutes of reaction, the pronounced surface functionalization is reflected by the Raman spectrum displayed in Fig. 1d . By a detailed line-shape analysis of the spectra, at least seven main features could be identified. The most prominent can be assigned to the graphitic E 2g G mode ( ∼ 1,575 cm −1 ), while we attribute the slight deviation in the phonon frequency to strain present in the GIC [21] . In addition to the well-known dispersive D mode ( ∼ 1,340 cm −1 ), five additional modes (D 1 –D 5 ) were identified for the first time. These modes are assigned as D 1 ( ∼ 1,325 cm −1 ), D 2 ( ∼ 1,442 cm −1 ), D 3 ( ∼ 1,483 cm −1 ), D 4 ( ∼ 1,518 cm −1 ) and D 5 ( ∼ 1,559 cm −1 ). Their appearance is based on the change of hybridization in the graphene lattice in close proximity to the hydrogenated carbon atoms. As will be demonstrated below ( Fig. 2c,d ) by a direct comparison with the results obtained by quantum mechanical calculations, these modes can be assigned to specific lattice vibrations. The pronounced C Z mode ( ∼ 560 cm −1 ), indicating graphitic intercalation architecture in the bulk crystal, is widely retained ( Fig. 1c ). On the other hand, the additional D modes clearly reflect the functionalization process on the surface. Mechanistically, a single electron transfer from the GIC to water protons and a subsequent addition of H-radicals to the oxidized graphene surface is assumed [7] , [21] . Both the presence of a C Z mode and the absence of any second-order mode in the final spectrum show that the GIC oxidation of the bulk crystal is not complete. Obviously, the oxidation potential of H 2 O and the limited mobility of K + in the inner part of the crystal are not sufficient enough to allow for a complete bulk reoxidation, but can be used for a surface or thin film functionalization. The reaction comes to an end when a limiting stoichiometry of n K + C 8 ( n - m )− H m is reached, as indicated in the spectrum presented in Fig. 1d . This in situ investigation of the reductive graphene functionalization process allowed for a clear identification and correlation of introduced sp 3 defect sites and related new Raman vibrational modes. 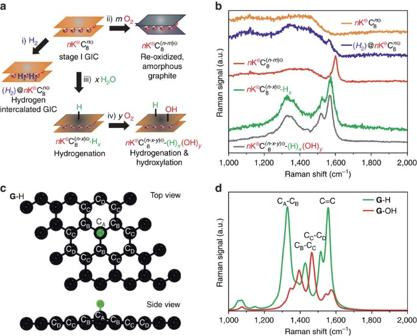Figure 2: Identification and assignment of new Raman bands in G-H. (a) Systematic study of KC8exposed to (i) hydrogen, (ii) oxygen and (iii) water that was subsequently exposed to (iv) oxygen. The correspondingin situRaman spectra are shown inb. Starting from saturation doped KC8, (i) H2leads to intercalation, (ii) O2to reoxidation to amorphous graphite and (iii) H2O tosp3defect site formation by hydrogenation. If (iv) O2is added in combination with H2O, also hydroxylation takes placed. (c) 4 × 4 supercell of 32 lattice carbon atoms with asp3C-H moiety attached to carbon atom CAand the directly neighbouring labelled lattice carbon atoms CBand CC. Reference supercells for defect-free grapheneG: seeSupplementary Fig. 5; supercells for hydroxylatedG-OH: seeSupplementary Fig. 6. (d) The calculated Raman spectra between 1,000 and 2,000 cm−1with one hydrogenated/hydroxylatedsp3carbon atom in a cell of 32 graphene lattice carbon atoms, respectively. For the detailed information on vibrational frequencies and a visualization of the modes seeSupplementary Tables 1 and 2. Figure 2: Identification and assignment of new Raman bands in G-H. ( a ) Systematic study of KC 8 exposed to (i) hydrogen, (ii) oxygen and (iii) water that was subsequently exposed to (iv) oxygen. The corresponding in situ Raman spectra are shown in b . Starting from saturation doped KC 8 , (i) H 2 leads to intercalation, (ii) O 2 to reoxidation to amorphous graphite and (iii) H 2 O to sp 3 defect site formation by hydrogenation. If (iv) O 2 is added in combination with H 2 O, also hydroxylation takes placed. ( c ) 4 × 4 supercell of 32 lattice carbon atoms with a sp 3 C-H moiety attached to carbon atom C A and the directly neighbouring labelled lattice carbon atoms C B and C C . Reference supercells for defect-free graphene G : see Supplementary Fig. 5 ; supercells for hydroxylated G -OH: see Supplementary Fig. 6 . ( d ) The calculated Raman spectra between 1,000 and 2,000 cm −1 with one hydrogenated/hydroxylated sp 3 carbon atom in a cell of 32 graphene lattice carbon atoms, respectively. For the detailed information on vibrational frequencies and a visualization of the modes see Supplementary Tables 1 and 2 . Full size image Reaction of GICs with hydrogen or oxygen and water In another series of experiments we addressed the question of how GICs respond to the exposure of H 2 , O 2 and a combination of O 2 and H 2 O to simulate their behaviour under ambient conditions. The corresponding results are depicted in Fig. 2 . We expected that KC 8 should not give rise to covalent hydrogenation with H 2 gas under these conditions [37] . Indeed, as can be seen in Fig. 2b , H 2 exposure does not yield any covalent binding to the graphene lattice since the Fano-shaped signature of stage I GICs is largely preserved ( Fig. 2b , blue). The corresponding evolution of the Raman spectra ( Supplementary Fig. 2a ) rather indicates H 2 intercalation, leading to (H 2 )@ n K + C 8 n − . The intercalation of H 2 in between the graphene sheets is clearly corroborated by an increasing intensity of the C Z mode. In addition, the exclusive exposure of oxygen gas to the GIC was also studied ( Supplementary Fig. 2b ). The evolution of the Raman spectra clearly underlines that pure oxygen is not covalently reacting with KC 8 but leads to a partial oxidation with the result of a lower overall potassium loading. This can be clearly recognized from the final Raman spectrum in Fig. 2b (red), where no defect site-related fingerprint was observed. We assume that exposure of KC 8 to O 2 leads to the formation of potassium superoxide [1] , [14] . Hence, the reoxidation by oxygen without mass transport of potassium (in contrast to, for example, the oxidation in benzonitrile [6] ) leads to disordered graphite that is clearly revealed in the respective XRD pattern ( Supplementary Fig. 3 ). To simulate ambient workup conditions with our setup, first the same hydrogenation reaction as shown in Fig. 1 was initiated, leading to partially reoxidized and covalently hydrogenated n K + C 8 ( n - m )− H m . Subsequently, the sample was exposed to oxygen in the presence of water. Under these conditions the material should be reoxidized and simultaneously a hydroxylation of the carbon scaffold can be expected [14] . This formation of -OH entities in the presence of oxygen and water has recently been confirmed for graphenide solutions [6] and therefore represents a major field of interest in reductive functionalization of carbon allotropes. The in situ Raman analysis in Fig. 2b clearly revealed that in this case further covalent binding is promoted. It can be assumed that after the initial treatment with H 2 O vapour, a water film is still absorbed on the graphitic surface. Subsequent single electron transfer processes between the GIC and O 2 can now be accompanied by follow-up reactions with H 2 O. In the Raman spectra this is reflected by an additional defect site-related interband appearing at 1,460 cm −1 . This mode can be assigned to C-O vibrations that relate to the functionalization with covalently sp 3 bound -OH groups. In agreement with literature, this Raman fingerprint has already been predicted by theory [22] and investigated for graphene oxide [27] . Importantly, our present study can unambiguously verify the proposed origin of this band by theoretical calculations ( Fig. 2d ) and by temperature-dependent Raman spectroscopy (TDRS) in combination with TG-MS (thermogravimetric analysis coupled to mass spectrometry) analysis ( Supplementary Fig. 4 ). These findings prove that the covalent hydroxylation of graphenide requires the presence of both oxygen and water [6] that are omnipresent under ambient conditions. Hence, the sole treatment with oxygen is not sufficient, strongly supporting the reported mechanism for the hydroxyl functionalization [14] . Calculation of the vibrational Raman response To address the lattice carbon bond vibrational coupling deviation from the normal E 2g G mode related to the C=C sp 2 vibrations in graphene at ∼ 1,580 cm −1 upon introduction of sp 3 defect sites and the corresponding additional C-C modes, the vibrational Raman response of pristine graphene functionalized by either a hydrogen or hydroxyl addend was calculated. Therefore, a 4 × 4 supercell of graphene (32 lattice carbon atoms) functionalized with one -H or -OH moiety (3.125% DOF) was considered ( Fig. 2c ). The addend carrying sp 3 hybridized lattice carbon atom is labelled C A , while the direct neighbouring basal C atoms are termed C B and those next to it C C and C D . The resulting calculated Raman spectra for hydrogenated G -H and hydroxylated G -OH are presented in Fig. 2d , respectively. The simulated reference for defect free graphene G is provided in Supplementary Fig. 5 . With respect to the approximations made in the calculations, the limitations provided by the experimental setup (resolution of the detector and calibration ambiguity) and the fact that the covalently functionalized graphene sample is a mixture of hydroxylated and hydrogenated species with varying content, the calculated and experimental values for the evolving bands is in good correlation. In the case of G -H the hybridization change is accompanied by lifting the hydrogenated C-atom by ∂ z =0.46 Å out of plane in z -direction ( Fig. 2c ). Along with this shift, the C B –C A –C B dihedral angle changes from γ =120° (pure sp 2 in pristine graphene) to γ =114.5° for G -H ( Supplementary Fig. 7a ) and to γ =113.7° for G -OH ( Supplementary Fig. 6a ). The complete list of calculated angles, shifts and phonon frequencies is provided in Supplementary Table 1 . The theoretical analysis provides the phonon energy for excitations of lattice carbon atoms surrounding a sp 3 defect is affected by the newly formed C-H bond. The geometry around the C-H/ sp 3 centre ( γ (C B C A C B )=114.5°) is strained, since it deviates from the regular tetrahedral angle of 109.5°. The appearance of the additional D 1 –D 5 modes between 1,300 and 1,600 cm −1 is a consequence of these new geometrical constraints. When the DOF is increased, structures of curved nanodiamond clusters are eventually emerging strongly reassembling the Raman spectra of n K + C 8 ( n - x )− -H x and n K + C 8 ( n - x-y )− (H) x (OH) y in Fig. 2b (ref. 38 ). These findings are fundamental for the general interpretation of the Raman spectra of any covalent graphene derivative, since the broadening of the modes can now be precisely attributed to distinct vibrations. These results are in line with previous reports on the clustering of defect centres upon increasing the DOF [39] , [40] , [41] , [42] , [43] , [44] . The newly observed D 1 –D 5 modes start appearing in the spectra only beyond a certain DOF ( θ < ∼ 0.5%). At even higher degrees of functionalization ( θ >3%), these modes broaden, causing a much less structured Raman spectrum, typically observed for highly functionalized graphene such as graphene oxide [34] , [45] . As a consequence, the resolution and assignment of the additional modes D 1 –D 5 reaches an optimum in a range of functionalization ( ∼ 0.5%< θ < ∼ 2%) corresponding to the in situ situation depicted in Fig. 4b . 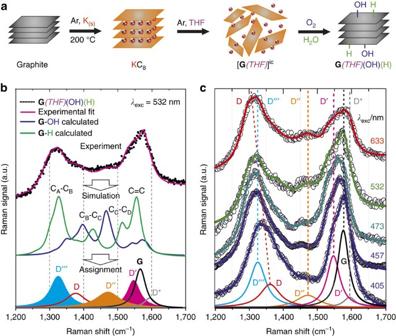Figure 3: Raman bands in bulk functionalized samples. Raman spectroscopy of a bulk functionalized graphene derivativeG(THF)(OH)(H) as a model of GO without σ-defects45. (a) Reaction scheme for the hydrogenation and hydroxylation of charged graphenides followed by workup under ambient conditions (O2/H2O). (b) Raman D- to G-mode area ofG(THF)(OH)(H) together with the corresponding calculated spectra forG-OH (blue) andG-H (green). The combination of experiment and theory leads to a precise assignment of each Raman mode. Besides the D, D* and G modes arising from excitations at theKpoint, the Raman fingerprint of covalently functionalized (here: -OH and -H) lattice carbon atoms can be revealed by identifying the modes D’’’, D’’ and D’. (c) Raman analysis with varying laser excitation wavelengths: 405 to 633 nm. Every mode but the D mode is nondispersive (excitation at theΓpoint) as expected in relation to the Raman fingerprint obtained inFig. 1. The determined Raman shifts for the individual components are summarized inSupplementary Table 1. Figure 3: Raman bands in bulk functionalized samples. Raman spectroscopy of a bulk functionalized graphene derivative G (THF) (OH)(H) as a model of GO without σ-defects [45] . ( a ) Reaction scheme for the hydrogenation and hydroxylation of charged graphenides followed by workup under ambient conditions (O 2 /H 2 O). ( b ) Raman D- to G-mode area of G (THF) (OH)(H) together with the corresponding calculated spectra for G -OH (blue) and G -H (green). The combination of experiment and theory leads to a precise assignment of each Raman mode. Besides the D, D* and G modes arising from excitations at the K point, the Raman fingerprint of covalently functionalized (here: -OH and -H) lattice carbon atoms can be revealed by identifying the modes D’’’, D’’ and D’. ( c ) Raman analysis with varying laser excitation wavelengths: 405 to 633 nm. Every mode but the D mode is nondispersive (excitation at the Γ point) as expected in relation to the Raman fingerprint obtained in Fig. 1 . The determined Raman shifts for the individual components are summarized in Supplementary Table 1 . 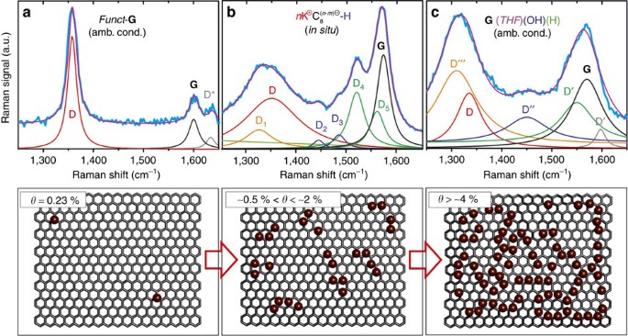Figure 4: Evolution of Raman fingerprint with increasing DOF. (a) Hexyl functionalized graphene10with isotropic distribution of functional groups with lateral DOF ofLD>2 nm (θ<0.5%). (b) Local clustering of defect sites as observed in thein situmonitoring of the functionalization in a typical range ofθ=0.5–2% using the precisely determined modes displayed inFig. 1d. (c) Higher DOF (θ>2%) resulting in isolatedsp2domains surrounded by defect-richsp3regions. Full size image Figure 4: Evolution of Raman fingerprint with increasing DOF. ( a ) Hexyl functionalized graphene [10] with isotropic distribution of functional groups with lateral DOF of L D >2 nm ( θ <0.5%). ( b ) Local clustering of defect sites as observed in the in situ monitoring of the functionalization in a typical range of θ =0.5–2% using the precisely determined modes displayed in Fig. 1d . ( c ) Higher DOF ( θ >2%) resulting in isolated sp 2 domains surrounded by defect-rich sp 3 regions. Full size image Raman assignment in highly functionalized graphene To further demonstrate the importance of this powerful characterization, we applied our Raman fingerprint assignment to crosscheck and analyse highly functionalized reaction products after workup. As a bulk functionalization approach we have chose the reaction of KC 8 dispersed in tetrahydrofuran (THF), resulting in the exfoliation of the graphenide sheets [ G (THF) ] ic ( Fig. 3a ) [2] , [3] . Before the functionalization step, we observed no indication that KC 8 would undergo any reoxidation or chemisorption within the dry solvent THF. For the covalent functionalization the intermediate [ G (THF) ] ic was subsequently exposed to oxygen and water. The resulting Raman spectrum of bulk functionalized powder sample after workup ( Fig. 3b ) resembles the typical Raman signature of GO where three broad overlapping modes are observed in the Raman shift regime between 1,200 and 1,650 cm −1 (ref. 22 ). In the double resonance area between 2,500 and 3,400 cm −1 , the three main components 2D, D+G and 2D* can be identified. So far, these features have neither been assigned to vibrations of specific addends nor have they been used to quantify the defects in GO. We show now that the deconvolution of such spectra ( Fig. 3b , top) can be accomplished and a detailed analysis of the structural composition can be provided. For this purpose the defect site-related Raman fingerprint with the characteristic modes termed as D′′′, D′′ and D′ were fitted to the spectrum in Fig. 3b . These modes are located at the same Raman shift positions as the previously determined interbands (D 1 –D 5 ) of the mildly functionalized charged graphite, generated in situ before workup, and can therefore also be precisely identified. As indicated in Fig. 4 the D 1 , D 2 /D 3 and D 4 /D 5 modes can be correlated with the D′′′, D′′ and D′ interbands. Consequently, these bands can be assigned to the calculated vibrational modes C A –C B (D 1 , D′′′), C B –C C (D 2 /D 3 , D′′) and C C –C D (D 4 /D 5 , D′), respectively ( Fig. 3b ). After complete reoxidation, the intravalley D* mode could be identified that cannot be observed in an intermediate charged state [7] , [21] . The interbands D 1 –D 5 of partial reacted graphene also vary in position and intensity in comparison with D′′′, D′′ and D′ of the completely reoxidized counterparts. For a better understanding of the correlation between the different labelling formats ( in situ , calculated, after workup) the respective information is summarized in Supplementary Table 1 . TDRS and thermogravimetric analysis For an independent chemical analysis of the nature of the grafted addends, TDRS was carried out and compared with the corresponding TG-MS results ( Supplementary Fig. 4 ). This correlation allowed for the unambiguous assignment of each component in the Raman spectra. Upon thermal defunctionalization, the defect-related Raman signatures vanish at the same temperature where the -H and -OH addends are cleaved [6] . The development of the individual peak intensities as a function of temperature is displayed in Supplementary Fig. 4b . In accordance with GO [27] ( Fig. 2d ), we observe a decrease of the oxygen-related D′′ mode (assigned by calculations) over the whole temperature range, while the remaining functionalities—mainly hydrogen—are cleaved at higher temperatures [31] , [32] . Remarkably, the evolution of this defect state-related Raman mode directly correlates with the thermal cleavage of the -OH addends ( m / z 17) determined by TG-MS ( Supplementary Fig. 4d ). Moreover, the dehydrogenation is clearly reflected by the m / z 2 trace between 350 and 600 °C. This thermal dehydrogenation is accompanied by a simultaneous decrease of the D′′, D′ and the D modes above 400 °C as depicted in Supplementary Fig. 4b . Multifrequency Raman analysis of the sample Finally, to further confirm the experimental assignment of the Raman modes, a multifrequency Raman study was conducted ( Fig. 3c ). Since our initial laser wavelength of 532 nm (2.33 eV) resulted in an exact superimposition of the nondispersive D′′′ mode excited at the Γ point of the Brillouin zone ( ∼ 1,325 cm −1 ) and the dispersive D mode from the K point ( ∼ 1,340 cm −1 ). To prove this assumption, we varied the excitation wavelength from 405 to 633 nm for highly functionalized samples as shown in Fig. 3c (ref. 15 ). Our results confirm the dispersion of the D mode in highly functionalized graphene and the nondispersivity of the D′′′ mode at ∼ 1,325 cm −1 . To double check the experimental assignments of each component, we carried out a cross-correlation employing the calculated Raman spectra of G -OH and G -H. Remarkably, this simulation fully matches the experimental Raman fingerprint as demonstrated in Fig. 3b . It has to be noted that for the calculation of the Raman modes, a 4 × 4 supercell was used. This scenario, however, does not reflect the Raman processes at the K point of the graphene Brillouin zone, preventing the simulation of the D and D* modes. Nevertheless, all other defect site-related Raman modes can be clearly assigned. The D-mode region is composed of two main components, as the nondispersive D′′′ mode and the dispersive D mode are superimposed for λ exc =532 nm. Moreover, the individual components of the Raman signal can be correlated with the TG-MS analysis ( Supplementary Fig. 4 ). Hence, this spectroscopic fingerprint is the first direct verification of the chemical nature of sp 3 defects (here: -OH and -H) present in the sample. The variation of the laser excitation energy proved that none of these modes are dispersive but the Raman D mode, entirely agreeing with our experimental and theoretical model of locally modified lattice carbon vibrations and molecular environments. In Fig. 4 , the Raman spectra of three samples exhibiting a different DOF are presented to demonstrate the evolution of the Raman signatures with increasing sp 3 carbon atom content. As an example of a graphene derivative with a very low DOF ( θ <0.5%), a typical Raman spectrum of a hexyl functionalized derivative, on which we reported previously [10] , is presented in Fig. 4a . This reductively functionalized sample has an isotropic distribution of defects with a distance of L D >2 nm, resulting predominantly in the activation of the D and D* mode in the Raman spectrum. In this simple case, the I D / I G ratio can be used for the determination of θ (ref. 9 ). In this case, the narrow width of the D mode (22 cm −1 ) relates to θ =0.23%. At such low densities of defects, no additional Raman modes can be deduced and the deconvolution into D, G and D* modes can be easily carried out. This is in very good agreement with the observed maximum in the D/G ratio in defective graphene and graphite at L D of ∼ 3 nm (ref. 28 ) and 4 nm (ref. 29 ), respectively. The deconvolution of these modes becomes more challenging if the DOF is further increased, as the D/G ratio is reduced concomitant to a line broadening [28] , [29] . Our results allow to clearly attribute the origin of this broadening to the additional evolving Raman interband modes. For clarity, the Raman spectrum of functionalized graphene with θ =1.6% is shown in Supplementary Fig. 8a . With ongoing functionalization, monitored by the laser probe, similar Raman interbands termed D 1 –D 5 are revealed in the in situ reaction of KC 8 with H 2 O (compare Fig. 4b ). The DOF of this in situ resolved state can be attributed to a range of θ =0.5%< θ <2%. In the corresponding covalent adducts the addends are already clustered within sp 3 defect site regions, although >98% of the basal carbon atoms are still intact. The cartoons in Fig. 4 are presented to visualize the relationship between the observed Raman interbands and the respective structure on the graphene sheet. Upon approaching the maximum DOF after full reaction of KC 8 under ambient conditions ( Fig. 4c ), GO with θ =6.0% serves as ideal reference [22] , [27] , since the Raman modes do not change their shape but their overall intensity [30] ( Supplementary Fig. 8b ). Thus, the analysis of all assigned Raman interbands, both in GO and in G (THF) (OH)(H) ( Fig. 3a ), allows for the characterization of adducts with θ >2%. In this range, all additional components (D′′′–D′) in the Raman spectrum are clearly identifiable. The observed fingerprint fully matches the simulated spectra for G -H and G -OH ( Fig. 3d ) that were also calculated for θ ≈3%. This is in full agreement with recent surface-enhanced Raman scattering studies on functionalized chemical vapour deposition graphene, where a slight fingerprint for chemically modified graphene with a DOF of ∼ 0.5% leads to comparably weak Raman interbands in the D- and G-mode area [46] . Thus, we can conclude that the approach towards the maximal possible DOF of 12.5% (based on the ratio of K/C=1:8) is accompanied by clustering of addends and by the formation nonaltered sp 2 nano domains [39] , [40] , [41] . In summary, we report a comprehensive study involving in situ Raman spectroscopy supported by quantum mechanical calculations to exactly monitor the covalent binding to graphene with unprecedented precision. This approach is very general and also allows for the fast screening and evaluation of suitable reaction conditions for covalent graphene functionalization. As model reaction we have chosen the hydrogenation of reduced graphite (KC 8 ) with H 2 O and compared it with the corresponding exposure to H 2 and O 2 . The early stages of graphene hydrogenation are accompanied by the evolution of a series of so far undiscovered D-modes (D 1 –D 5 ). Using quantum mechanical calculations we were able to unambiguously assign these bands to distinct lattice vibrations in the neighbourhood of the covalently bound addend. Interestingly, the exposure of KC 8 to H 2 and O 2 did not cause covalent binding but intercalation of molecular H 2 or partial oxidation, respectively. A combination of H 2 O and O 2 treatment led to the formation of additional hydroxyl (-OH) functionalities that were clearly identified by Raman spectroscopy and TG-MS. The latter reaction represents a very suitable model for the decomposition of graphenides under ambient conditions (hydrogenation and hydroxylation). This important process has so far never been analysed in detail. We have further demonstrated that our fundamental mechanistic investigation brings us into the position to simulate and assign the spectroscopic signatures of both bulk functionalized G (THF) (OH)(H) and GO [34] . Finally, we have also applied our concept to simulate and characterize additional covalently functionalized graphene derivatives prepared as bulk materials with different composition (for example, DOF and nature of covalent addend) demonstrating the generality of the method. So far, covalent graphene functionalization remained a very difficult field of synthetic chemistry. This is not only because suitable methods enabling graphite/graphene activation and dispersion had to be identified to allow an efficient adduct formation. A major challenge was also the satisfactory characterization of reaction products since the typical powerful tools applied in synthetic chemistry such as nuclear magnetic resonance spectroscopy and mass spectrometry cannot be applied to this polydisperse 2D material. In this regard, the work presented here is a major breakthrough as it allows for graphene-derivative characterization with unprecedented precision. Raman spectroscopy In situ Raman spectroscopic detection was carried out inside a quartz tube through a flat (0.7 mm thick) optical window of borosilicate glass (PGO GmbH) in ultra-high vacuum chamber at ∼ 4 × 10 −8 mbar where the intercalated GIC was placed in a sample boat. The Raman measurements were performed at room temperature using a HORIBA LabRam spectrometer with a 514 nm excitation wavelength at 0.5 mW between 300 and 3,000 cm −1 . To avoid laser-induced deintercalation and photochemistry, the laser power was kept below 0.5 mW. The Raman spectroscopic characterization of samples exposed to ambient conditions and workup was carried out on a Horiba Jobin Yvon LabRAM evolution confocal Raman microscope (excitation wavelengths: 405, 457, 473, 532 and 633 nm) with a laser spot size of ∼ 1 μm (Olympus LMPlanFl 50 × , NA 0.50). Raman measurements were carried out using a micro-Raman setup in backscattering geometry. A charge-coupled device is used to detect the signal after analysing the signal via a monochromator. The spectrometer was calibrated in frequency using a HOPG crystal. Thermogravimetric analysis and mass spectrometry For G -H and G -OH, the TG-MS analyses was carried out on a Netzsch STA409 CD instrument equipped with a Skimmer QMS 422 mass spectrometer (MS/EI) with the following programmed time-dependent temperature profile: 30–700 °C with 20 K min −1 gradient and cooling to 30 °C. The initial sample weights were adjusted at 5.0 (±0.1) mg and the whole experiment was executed under inert gas atmosphere with a He gas flow of 80 ml min −1 . The obtained data were processed with the Netzsch Proteus Analysis software. X-ray diffraction XRD was performed by placing the material in a glove box into glass capillaries with 1.5 to 2 mm diameter and 10 μm wall thickness (Hilgenberg, Germany) and subsequent sealing. X-ray patterns were measured using a microfocus X-ray source with a copper target ( λ =1.542 Å) equipped with a pinhole camera (Nanostar, Bruker AXS) and an image plate system (Fujifilm FLA 7,000). All two-dimensional WAXS patterns were radially averaged and background corrected to obtain the scattering intensities in dependence on the scattering angle 2 θ . Glovebox Sample preparation, solvent processing and bulk functionalization were carried out in an argon-filled Labmaster SP glovebox (MBraun), equipped with a gas filter to remove solvents and an argon cooling systems, with an oxygen content <0.1 p.p.m. and a water content <0.1 p.p.m. Graphite As starting material a spherical graphite SGN18 (Future Carbon, Germany), a synthetic graphite (99.99% C, <0.01% ash) with a comparatively small mean grain size of 18 μm ( Supplementary Fig. 9 ), a high specific surface area of 6.2 m 2 g −1 and a resistivity of 0.001 Ω cm was chosen. An average Raman I D / I G intensity ratio of 0.3 is present in the starting material ( Supplementary Fig. 10 ). Potassium chunks Potassium was bought from Sigma-Aldrich Co. and used as received (99.99% purity). Oxygen 4.5 (O 2 ) and hydrogen 5.0 (H 2 ) The gases used for the functionalization were received as lecture gas bottles (Minican) from Linde and directly connected to the in situ Raman measurement setup. Water (H 2 O) Water was received from Sigma-Aldrich purified, deionized and bidistilled. Pump-freeze technique was carried out 3 times to completely remove gases from the water. Tetrahydrofuran THF was received anhydrous from Sigma-Aldrich Co. and dried over molecular sieves (3 Å). Subsequently, it was distilled over Na/K alloy to remove inhibitor and achieve absolute quality (<1 p.p.m. H 2 O, <1 p.p.m. O 2 ). Finally, pump-freeze technique was used to completely degas the solvents before the reaction. Preparation of K 8 C graphite intercalation compound For the synthesis of solid-state GIC mother batch, 480 mg (40 mmol carbon) spherical graphite SGN18 and 195 mg (5 mmol) potassium were heated to 200 °C in a glass vial in the glovebox. The formation of the final-stage I intercalation compound was verified by in situ Raman spectroscopy ( Fig. 1c ) and XRD analysis ( Supplementary Fig. 1 ) under inert conditions, respectively. After the complete formation of the stage I K GIC, the powder was allowed to cool to ambient temperature and evacuated to ultra-high vacuum conditions before the reoxidation experiments carried out in the in situ spectroscopy setup. Controlled functionalization of the graphite intercalation compounds The vapour pressure controlled exposure of the GIC towards H 2 O, O 2 and H 2 was carried out in the specialized setup in Fig. 1a . To achieve an efficient monitoring of the reaction between KC 8 and the respective reagent, the reservoir valve was opened until the pressure in the chamber was raised from 10 −8 to 10 −5 mbar. To further increase the concentration of reagent we stepwise allowed an increase to normal pressure for a complete floating of the sample by the reagent. Functionalized bulk sample preparation and workup Workup of the samples at ambient conditions ( Fig. 3 ) for the synthesis of G (THF) (OH)(H): for the Raman analysis after workup, 5 mg of KC 8 was dispersed in purified THF and subsequently exposed to oxygen and water under ambient conditions. After 1 h of reaction time, the black powder was washed with 10 ml of cyclohexane, ethanol and water to remove salts and solvent residues, respectively. For the final Raman analysis, the sample was dried at 70 °C overnight. The functionalized graphene derivatives funct - G ( Fig. 4 and Supplementary Fig. 8a ) as well as GO were produced, characterized and fitted according to literature [30] . Experimental details for the synthesis of the functionalized graphene derivatives aryl- G : Bis-(4- tert -butylphenyl) iodonium hexafluorophosphate was deposited from solution (CH 2 Cl 2 ) on monolayer graphene ( Supplementary Fig. 8 ). The reaction of 4- tert -butylphenyl ( t BP) cations was subsequently activated by a laser pulse (532 nm, 5 s, 10 mW) within the Raman spectrometer. GO with DOF θ =6.0% was synthesized with graphite sulfate as starting material [47] . Computational details Density-functional calculations were carried out with the Vienna ab initio Simulation Package (VASP) [48] that employs a plane-wave basis set. We have used ‘hard’ pseudopotentials with a smaller core region to allow for more flexibility in the description of the valence electrons. The exchange–correlation functional due to Perdew–Burke–Ernzerhof was employed [49] . An energy cutoff of 600 eV was used. Electronic structures and geometries were converged below 1 × 10 −8 eV and 0.001 eV Å −1 with respect to total energies and forces acting on ions, respectively. We have applied a slab approach with vacuum layers of 15 Å to decouple periodic images from each other along the z direction. The Brillouin zone was sampled by 5 × 5 × 1 Monkhorst–Pack K- point grids [50] for hexagonal (4 × 4) unit cells with 32 carbon atoms. Vibrational frequency calculations were performed using the finite difference method. Raman intensities are calculated from the change in polarizability upon following the Eigen mode of the phonon [51] . This is calculated using the finite difference method with backward and forward calculations of each Eigen mode displacement. The dielectric tensor is reduced to a scalar in the far-from-response Raman approximation. The Γ point-centred phonon modes weighted by the computed spectral intensity convolved with a Gaussian function with a full width at half maxima of 5 cm −1 applied to all frequencies (for comparison with experimental results), as shown in Supplementary Figs 5–7 . Visualization of the calculated frequencies was performed using QVibeplot [52] . Data availability The authors declare that the data supporting the findings of this study are available within the article and its Supplementary Information Files . All other relevant data supporting the findings of this study are available from the corresponding author on request. How to cite this article: Vecera, P. et al . Precise determination of graphene functionalization by in situ Raman spectroscopy. Nat. Commun. 8, 15192 doi: 10.1038/ncomms15192 (2017). Publisher’s note: Springer Nature remains neutral with regard to jurisdictional claims in published maps and institutional affiliations.